Engineering fluid flow using sequenced microstructures Controlling the shape of fluid streams is important across scales: from industrial processing to control of biomolecular interactions. Previous approaches to control fluid streams have focused mainly on creating chaotic flows to enhance mixing. Here we develop an approach to apply order using sequences of fluid transformations rather than enhancing chaos. We investigate the inertial flow deformations around a library of single cylindrical pillars within a microfluidic channel and assemble these net fluid transformations to engineer fluid streams. As these transformations provide a deterministic mapping of fluid elements from upstream to downstream of a pillar, we can sequentially arrange pillars to apply the associated nested maps and, therefore, create complex fluid structures without additional numerical simulation. To show the range of capabilities, we present sequences that sculpt the cross-sectional shape of a stream into complex geometries, move and split a fluid stream, perform solution exchange and achieve particle separation. A general strategy to engineer fluid streams into a broad class of defined configurations in which the complexity of the nonlinear equations of fluid motion are abstracted from the user is a first step to programming streams of any desired shape, which would be useful for biological, chemical and materials automation. Control of fluid streams is useful in biological processing [1] , [2] , [3] , chemical reaction control [4] , [5] , and creating structured materials [6] , [7] , [8] ; however, general strategies to engineer the cross-sectional form and motion of fluid streams have been limited. Strategies to mix fluids [1] , [9] , [10] and control particles [11] , [12] using engineered systems exist, often relying on chaotic fluid transformations as an effective tool [13] , [14] to disrupt sustained regions of order in the flow [10] , [15] . Rather than apply flow transformations to prevent order, here we develop a hierarchical approach to engineer fluid streams into a broad class of complex configurations. The cross-sectional shape of a fluid is sculpted using the integrated inertial flow deformations induced by sequences of simple microstructures (that is, pillars) at a set of discrete locations within the channel cross-section. Importantly, each pillar-induced transformation is numerically simulated only once to achieve the net transformation that can be used in an arbitrary sequence. Discretization of single-pillar operations followed by their engineered superposition allows the hierarchical assembly of complex flow configurations, resulting in engineered cross-sectional shapes such as various concavity polygons, closed rings and inclined lines. The introduction of a general strategy to sculpt fluid streams in which the complexity of the nonlinear equations of fluid motion are abstracted from the user is the first step in being able to sculpt any flow shape of interest. Such a capability has broad implications: in biological sciences it can aid in sample preparation of cells by moving them into a wash solution for analysis without background, in analytical chemistry such an approach can tune the contact between fluid and structures to aid or prevent reactions, binding or heat transfer at a surface, and in materials science it allows sculpting of the full three-dimensional shape of polymerized fibres and particles for barcoding or self-assembly. Inertial flow deformation We use cylinders placed at various cross-stream locations of a channel as the fundamental operators for our flow sculpting scheme ( Fig. 1a ). These geometric obstacles can be used to induce significant deformations in flow, creating useful net rotational secondary flows that locally move and deform fluid parcels. Notably, this net twisting of fluid around a pillar has been neglected in microfluidic systems because fluid inertia is often not important in a wide range of conventional microfluidic flow conditions [16] . Flow around a pillar in a straight channel without inertia (that is, Stokes flow) requires fore-aft symmetry because of the mirror-symmetry of the flow upon time-reversal of the linear equations of motion [17] . Therefore, any secondary fluid motion directed within the channel cross-section [18] is completely reversed after passing the cylinder mid-plane. 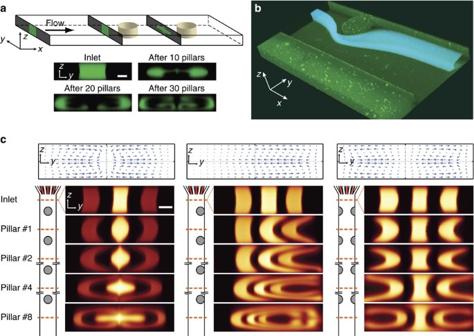Figure 1: Local inertial flow deformation induced by microstructures. (a) Flow passing a microstructure deforms significantly creating anetrecirculating secondary flow in the channel. The experimental results show the deformed stream, confirming the numerical prediction of net recirculating secondary flow. Scale bar, 25 μm. (b) A three-dimensional confocal microscopy image of a fluorescent stream deforming around a single-pillar in the channel clearly shows how the stream of fluid (sandwiched between the two streams of unlabelled fluid) is irreversibly twisted losing fore-aft symmetry around the pillar. The surface of the channel is labelled for a more vivid observation. (c) Position of the net circulation is controlled by pillar location. The top row shows the net deformation arrow plots for different pillar locations as predicted by numerical simulations. Below are the confocal images of channel cross-sections for each of the sequenced configurations. The lateral placement of pillar sequences is shown in the schematic. Three-labelled streams are tracked for a more detailed observation. By displacing the pillar centre from the middle to the side of the channel (left, middle, and right), the lateral position of the net recirculating flow is similarly displaced. All experiments are conducted atRe=20. Scale bar, 25 μm. Figure 1: Local inertial flow deformation induced by microstructures. ( a ) Flow passing a microstructure deforms significantly creating a net recirculating secondary flow in the channel. The experimental results show the deformed stream, confirming the numerical prediction of net recirculating secondary flow. Scale bar, 25 μm. ( b ) A three-dimensional confocal microscopy image of a fluorescent stream deforming around a single-pillar in the channel clearly shows how the stream of fluid (sandwiched between the two streams of unlabelled fluid) is irreversibly twisted losing fore-aft symmetry around the pillar. The surface of the channel is labelled for a more vivid observation. ( c ) Position of the net circulation is controlled by pillar location. The top row shows the net deformation arrow plots for different pillar locations as predicted by numerical simulations. Below are the confocal images of channel cross-sections for each of the sequenced configurations. The lateral placement of pillar sequences is shown in the schematic. Three-labelled streams are tracked for a more detailed observation. By displacing the pillar centre from the middle to the side of the channel (left, middle, and right), the lateral position of the net recirculating flow is similarly displaced. All experiments are conducted at Re =20. Scale bar, 25 μm. Full size image Unlike the fluid motion that completely reverses upon passing a micro-pillar for Stokes flow, flow with finite inertia is accompanied by a net deformation of fluid streams. Numerical simulations predict that as fluid passes through the centrally positioned pillars in a straight microchannel, the flow deforms in such a way that the fluid parcels near the channel centerline move outwards towards the side walls, while fluid parcels near the top and bottom walls move towards the channel centre ( Supplementary Fig. S1 ). This phenomenon, validated experimentally ( Supplementary Fig. S2 , Fig. 1 ), effectively creates a set of net rotational secondary flows within the microchannel ( Fig. 1a , Methods, Supplementary Movie 1 ). As a result, the flow is irreversibly twisted, losing its fore-aft symmetry near the pillar and causing a significant final deformation of the flow stream ( Fig. 1b ). The phenomenon has features in common with the secondary flow created in curved channels with finite inertia (Dean flow) [1] , [19] , [20] . In contrast with Dean flow, the lateral position of the pillar can be used to tune where the net recirculating flows are created across the channel ( Fig. 1c , Supplementary Fig. S3 ). By moving the sequence of pillars across the channel (in the y-direction) the centre of motion follows. This positioning enables spatial control over the induced deformation. For instance, by replacing the central pillars ( Fig. 1c left) with pairs of side half-pillars ( Fig. 1c right) the direction of the inertial flow deformation is reversed. The majority of the induced deformation occurs within four pillar diameters of the pillar for our flow conditions, prescribing an effective spacing between pillars for which the transformation from each individual pillar of a sequence behaves independently. Numerical comparison of Stokes and inertial flow development along the channel near the pillar indicates that the presence of the pillars leads to deformation of streamlines and while this deformation possesses fore-aft symmetry in Stokes flow, in agreement with the mirror-symmetry time-reversal theorem [17] , the symmetry is broken in the presence of inertia ( Fig. 2a ). Upstream, the inertial flow does not diverge greatly compared with Stokes flow. The two flows nearly match at x =0 (that is, the position of the pillar centre), while downstream of the pillar the inertial flow diverges greatly from Stokes flow creating a large deformation compared with the fluid topology at the inlet (that is, upstream of the pillar). This turning motion stops and flow deformation saturates ~3–4 pillar diameters downstream, such that we set an inter-pillar spacing of ten pillar diameters to ensure that when placed in a sequence the downstream flow profile of a previous pillar did not interact with the upstream profile of the next pillar. In this way the transformations performed by each pillar could be sequentially applied, without cross-talk between the independent operations, which would require fluid dynamic simulation of the combined sequence. 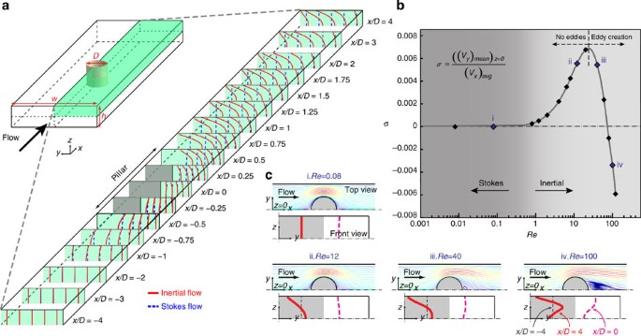Figure 2: Development of inertial flow deformation and operating regime. (a) Comparison of Stokes and inertial flow development along the channel near the pillar (shown in the top-right quarter of the channel). In each cross-section, using numerical simulations, we follow five vertical lines of tracer fluid parcels as they move past the obstacle and reach a stable state. The fore-aft symmetry of deformation that exists in Stokes flow is broken in the presence of inertia. (b) The graph showsσ, a measure of flow deformation away from the middle of the channel atz=0 over a wide range ofRe. (c) A more detailed simulation of a vertical set of inlet streamlines and their deformation in a quarter of the channel is provided for four differentRe. The top-view of streamlines atz=0 reveals the creation of post-pillar eddies with increasingRe,which corresponds to the shift from increasing to decreasingσwithRe. The front view illustrates the outline of an initially vertical line of fluid parcels at the inlet (dashed grey line), traced atx=0 (dashed pink line) and the outlet (solid red line). Solid black lines show channel walls and the dash-dot black lines indicate channel symmetry. The grey area shows the outline of a quarter of the pillar in the respective channel quarter. Figure 2: Development of inertial flow deformation and operating regime. ( a ) Comparison of Stokes and inertial flow development along the channel near the pillar (shown in the top-right quarter of the channel). In each cross-section, using numerical simulations, we follow five vertical lines of tracer fluid parcels as they move past the obstacle and reach a stable state. The fore-aft symmetry of deformation that exists in Stokes flow is broken in the presence of inertia. ( b ) The graph shows σ , a measure of flow deformation away from the middle of the channel at z =0 over a wide range of Re . ( c ) A more detailed simulation of a vertical set of inlet streamlines and their deformation in a quarter of the channel is provided for four different Re . The top-view of streamlines at z =0 reveals the creation of post-pillar eddies with increasing Re, which corresponds to the shift from increasing to decreasing σ with Re . The front view illustrates the outline of an initially vertical line of fluid parcels at the inlet (dashed grey line), traced at x =0 (dashed pink line) and the outlet (solid red line). Solid black lines show channel walls and the dash-dot black lines indicate channel symmetry. The grey area shows the outline of a quarter of the pillar in the respective channel quarter. Full size image The relatively uniform behaviour of inertial flow deformation over a range of flow rates in finite-Reynolds number laminar flows is an important feature for sculpting flow shapes over a range of conditions. The Reynolds number is a ratio of inertial to viscous forces in the flow ( Re=ρUH/μ ; here, H is the hydraulic diameter of the channel, U is the mean downstream velocity of a fluid with density ρ and viscosity μ) . We define σ to measure the magnitude of flow deformation away from the middle of the channel at z =0 (Methods). σ remains nearly uniform over an order of magnitude of Reynolds numbers (for Re ~6–60 ( Fig. 2b ), varying only by a factor of 2–3. Furthermore, while the net secondary flows behave consistently over a wide range of flow rates with a single-pillar diameter, σ was found to be tunable by adjusting the pillar diameter ( Supplementary Fig. S4 ). A closer examination of flow as a function of Re ( Fig. 2c ) reveals that for small channel Reynolds numbers, the flow behaves similar to Stokes flow, with no discernible flow deformation ( Re =0.08). Other methods to deform flow using structured channels [9] may be complementary for these conditions, however, these approaches operate less effectively as Re increases. In contrast, for the cylinders used here, as Re increases significant inertial flow deformation is observed ( Re =12). Increasing Re further leads to boundary layer separation along the downstream surface of the pillar and creation of post-pillar wake regions ( Re =40) in which the inertial flow deformation starts to manifest more complex behaviour ( Re =100). In this case, we observe that the fluid parcels near the top of the channel move towards the channel centre and that the flow starts to deform away from the channel centre further towards the z-mid-plane. Interestingly, the deformation is also directed towards the centre at z =0 ( Fig. 2c , Re =100). These results identify a range of flow conditions required to operate in a single mode but also suggest the ability to make use of separate modes of operation with more complex fundamental transformations over different flow conditions. Mode of flow deformation depends on system parameters Following the identification of this complexity in the single-pillar system, we systematically classified the range of possible flow deformations over the set of practically achievable controlling geometric and flow parameters. Dimensional analysis predicts that the behaviour of the system is described using three non-dimensional groups, for the case when the flow deformation-inducing obstacle is a cylinder at the centre of a straight channel: Re , channel aspect ratio h/w , and normalized pillar diameter D/w ( Fig. 3a ). For this case we uncover four dominant modes of operation for inertial flow deformation ( Fig. 3 ). The modes are defined based on the number of induced net secondary flows in a quarter of the channel (that is, one or two), as well as the direction of the net vorticity axis for each of these flows ( Fig. 3b ). Based on our numerical simulations we predict that four additional transitional modes of operation also exist, especially when pillar diameter is small ( Supplementary Fig. S5 ). However, for small D/w the net rotational flow remains weak ( Supplementary Fig. S4 ), such that these modes are not practically useful. Importantly, sensitivity analysis of the flow deformations around the pillars shows that they are stable in response to perturbations in system parameters such as channel geometry or flow conditions, with Reynolds number being the least sensitive parameter, and pillar projected diameter being the most sensitive ( Supplementary Note 1 , Supplementary Table S1 ). 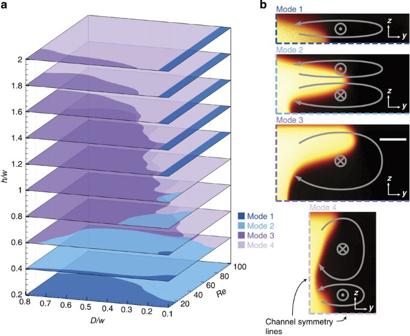Figure 3: Phase diagram for inertial flow deformation. (a) For the simplified case when the deformation-inducing obstacle is a cylindrical pillar at the centre of a straight channel, there are four dominant modes of operation. This phase diagram shows which mode is in effect at any given set of flow conditions and geometric parameters. (b) The four modes of operation achieved experimentally are shown with confocal cross-sections of the asymmetric quadrant of the flow (same scale bar of 20 μm is used for all four images). The images are overlaid with arrows indicating the direction of motion for that mode of operation. Figure 3: Phase diagram for inertial flow deformation. ( a ) For the simplified case when the deformation-inducing obstacle is a cylindrical pillar at the centre of a straight channel, there are four dominant modes of operation. This phase diagram shows which mode is in effect at any given set of flow conditions and geometric parameters. ( b ) The four modes of operation achieved experimentally are shown with confocal cross-sections of the asymmetric quadrant of the flow (same scale bar of 20 μm is used for all four images). The images are overlaid with arrows indicating the direction of motion for that mode of operation. Full size image Inertial flow deformation depends on gradients in fluid momentum and pressure across the channel cross-section that do not identically reverse fore and aft of the pillar. When there are no eddies present behind a pillar, the flow deformation occurring in this region dominates over the opposite-directed deformation occurring upstream of the pillar ( Fig. 2a ). We observe regions of lower pressure in the middle of the channel (due to the higher velocity fluid in this region) ( Supplementary Fig. S6 ), between two regions of high pressure on the top and bottom of the channel (near y =0). This leads to centre-directed motion of fluid parcels from the top and bottom of the channel, which is accompanied by movement of fluid parcels in the middle region to the sides, conserving mass (mode 1). However, increasing Re or changes in system geometry (for example, increasing channel aspect ratio) lead to creation of post-pillar eddies, which form a three-dimensionally complex closed region of recirculation behind the pillar ( Supplementary Fig. S7 ). This wake causes a reduction in the curvature for fluid streams transiting behind the cylinder and accompanying changes in the pressure field. The combination of these effects reduces the dominance of the deformation occurring downstream of the pillar, shifting the balance to the upstream deformation with net fluid rotation in the opposite direction, which corresponds to alternate modes of operation. Therefore, the motion is further complicated, in ways that we document with experiments and simulations useful for sculpting flow, by characteristics of flow past a bluff object, which includes the influence of boundary layer separation. Sequencing pillars to sculpt flow shapes The flow deformation operations we have demonstrated can be integrated to execute more sophisticated transformations and render complex flow shapes. We can numerically predict the inertial flow deformation near a single-pillar with high-precision ( Fig. 1c ). As discussed, if a set of pillars are appropriately spaced and sequentially placed along a channel, the output of each pillar can be taken as the input for the following pillar and the net deformation produced by the pillars can be combined sequentially. Therefore, by having the transformation function for a limited set of pillar configurations (that is, pillar size, lateral position), we can predict the total transformation function of any potential sequence, of which there are an infinite number ( Fig. 4a ). Consequently, a user can use a library of pre-simulated motions and place these in series to engineer a flow shape of interest quickly, at a low cost, with high accuracy and without any knowledge of fluid mechanics or numerical simulations. Systematic discretization of the pillar positions, similar to discretization of musical notes, allows abstraction and assembly of sequences, increasing the ability to engineer complex fluid systems ( Fig. 4b ). Therefore, each programme leading to an engineered flow shape is simply communicated using the inlet condition and the sequence of pillar positions ( Supplementary Fig. S8 ). For example, in Fig. 4ai an initially straight stream is transformed into a V-shape using the simple programme: c a b a c. The variety of attainable shapes include shapes with biconcave and biconvex areas ( Supplementary Fig. S8vii ), as well as closed loops ( Fig. 4aii ), sharp bends ( Fig. 4ai ), added vertices compared with the initial stream, and multiple changes in curvature ( Supplementary Fig. S8i, iii, vi ). 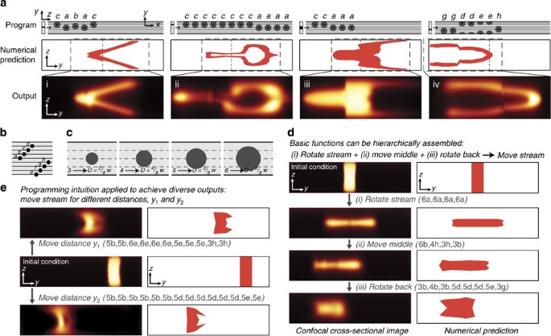Figure 4: Engineering fluid flow using programmed sequences of pillars. (a) Accurate numerical prediction of inertial flow deformation allows programming the cross-section of the flow. Each programme consists of (1) a sequence of pillars positioned at different locations across the channel, and (2) an initial condition, that is, inlet position and width of the fluid stream. The numerical predictions based on sequencing operations from a library of single-pillar flow transformation maps match very well with the experimental results. A user can use a library of pre-simulated motions and place these in series to engineer a flow shape of interest. (b) The systematic discretization of the pillar positions, similar to discretization of musical notes, facilitates the communication and reproducibility of different designs. (c) Systematic discretization of pillar sizes. (d) Hierarchical assembly of basic functions used to create a more complex operation. (e) Operations are performed on a single initial stream to achieve different outputs, for instance to move a single stream different distances across the channel. Figure 4: Engineering fluid flow using programmed sequences of pillars. ( a ) Accurate numerical prediction of inertial flow deformation allows programming the cross-section of the flow. Each programme consists of (1) a sequence of pillars positioned at different locations across the channel, and (2) an initial condition, that is, inlet position and width of the fluid stream. The numerical predictions based on sequencing operations from a library of single-pillar flow transformation maps match very well with the experimental results. A user can use a library of pre-simulated motions and place these in series to engineer a flow shape of interest. ( b ) The systematic discretization of the pillar positions, similar to discretization of musical notes, facilitates the communication and reproducibility of different designs. ( c ) Systematic discretization of pillar sizes. ( d ) Hierarchical assembly of basic functions used to create a more complex operation. ( e ) Operations are performed on a single initial stream to achieve different outputs, for instance to move a single stream different distances across the channel. Full size image There are, however, currently limitations to this technique. For instance, only shapes which have top–down mirror-symmetry are attainable, because of the symmetry of each individual flow transformation function. The area of the final shape is also constrained by conservation of mass, such that the velocity flux of the initial and final shape should be equal. This leads to the consequence that the cross-sectional flow shape area can either increase or decrease after the transformation, depending on whether the majority of fluid elements are nearer the slower moving channel wall or faster moving channel centerline. We also expect the final shape to be topologically simply connected without holes, although, practically, fluid splitting and enclosed regions can be achieved because diffusion also acts in the real system. Finally, the effect of pillars on coflowing streams cannot be easily decoupled, which means that it is best to engineer only one stream in a channel. Despite the limitations, this is an important step towards the ability to fully programme flow streams. As a result, analogous to software programming, a user can build upon previously demonstrated functions and integrate them in new ways to create more complex and useful outcomes. To expand the flow manipulation tool-box, the user can use various pillar diameters that enable finer control over strength and localization of the induced net secondary flows. Again, a discrete set of pillar sizes are coded to enable easy assembly as shown in Fig. 4c . For instance ‘ 6b ’ in a sequence indicates that the pillar diameter is 6 /8 of channel width ( Fig. 4c ), with its centre located at position b ( Fig. 4b ). Using a larger set of basic operations a user can engineer different flow manipulations more easily, for example, (i) rotate stream, (ii) move middle and (iii) rotate back, to achieve a more complex operation, such as moving a stream to one side of the channel ( Fig. 4d ). Although many of the design rules still need to be discovered, similar intuition developed by the designer for the assembly of complex functions at one location in a channel can be applied to different situations and inlet conditions. For instance a single stream can be moved to different lateral distances using the same design elements learned previously by one of the authors ( Fig. 4e ). The design elements used by the author can be described as follows: when operating in Mode 1, a pillar with its centre located near the centre of the stream of interest will push fluid in that stream outwards in the middle and inwards near top and bottom of the channel, an action which can be used to turn a vertical stream into a horizontal one (similar to Fig. 1c left for the middle stream). This can be followed by a sequence of pillars positioned asymmetrically on a side of the stream in order to then translate the previously positioned horizontal shape away from the positioned pillar (similar to Fig. 1c middle for a stream in the centre). Finally, the translated stream can be turned back to its vertical shape by using a sequence of pillars that are thoroughly off-centre from the stream (similar to Fig. 1c right for a stream near the channel centre). Applications of stream sculpting Taking advantage of the flow stream engineering capabilities, we apply inertial flow deformation to several example applications where lateral migration and manipulation of fluid streams or particles is required. We demonstrate fast and simple extraction of neutrally buoyant particles from a fluid stream ( Fig. 5a ), as well as particle separation and sorting by size ( Fig. 5b ), which are both useful operations to prepare cellular samples for downstream analysis. In these applications we also simultaneously make use of inertial focusing of particle streams that is dependent on particle size [11] , [16] , [21] . In this case while 10 μm particles maintain their preferred inertial focusing position due to larger inertial lift forces, smaller 1 μm particles or dye molecules, which experience two orders of magnitude weaker inertial lift forces, follow the flow streamlines away from the channel centre. More sophisticated sequences of pillars enable cross-stream translation of a fluid stream and solution exchange around particles in which both the particles and fluid stream stay focused ( Fig. 5c ). The preliminary results for solution exchange with this platform reach the highest achievable throughputs for cell separation compared with other state of the art techniques (~30–40 μl min −1 for the cell stream) [22] , [23] . Performance of these systems is also comparable: By using our engineered sequence of pillars operating at 250 μl min −1 upstream of a 7-fraction outlet (where the fluidic resistance of outlet fractions were designed to result in a specific distribution of outflow in each fraction), we were able to capture 96.0% (CV=14.6%) of 10 μm particles with a low contamination of background solution (10.8%, CV=0.19%) in outlet fraction 4, while recapturing a total of 83.8% (CV=0.20%) of the bead-free solution with only 3.85% (CV=0.10%) bead contamination in outlet fractions 5 and 6. Inertial flow deformation can also be used to split a single stream at the inlet into two or three streams across the channel, which can be useful in parallelization of screening applications such as flow cytometry ( Fig. 5d ). In the previous example, channel expansion allows multiple pillars to simultaneously perform operations on different pieces of the flow stream. Finally, the strong deformations create a semi-helical motion in the flow, which can be used to enhance mixing at high Peclet numbers ( Fig. 5e ). For this non-optimized case of only centrally located pillars, full mixing is achieved at high flow rate ( Pe ~4 × 10 4 ) in >3 cm, comparable with previous optimized mixers [9] ( Pe ~2 × 10 5 ), which normally operate at much smaller Re ( Re <0.1). Overall, many of the presented applications are best performed at either high rates to increase throughput, high Reynolds numbers to allow compatibility with inertial control of particles, or high Peclet numbers to prevent diffusive blurring of a sculpted material shape, such that the current approach that operates effectively outside of a Stokes flow regime is ideal. 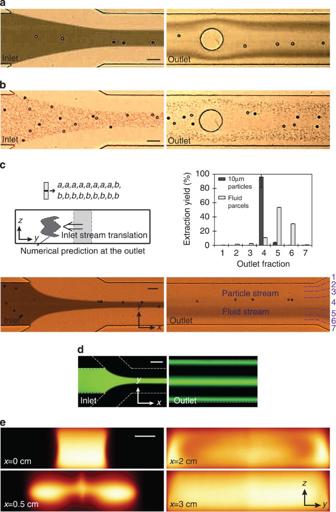Figure 5: Applications of fluid flow programming. (a) Extraction of particles from a fluid stream. While the fluid moves away from the channel centre due to inertial effects, particles are maintained at the channel centerline due to inertial focusing. (b) Separation of particles by size using a similar geometry (10 μm particles remain focused while 1 μm particles follow fluid streams). (c) Moving fluid streams and solution exchange around particles. High extraction yield (>95%) with high purity (>90%) is achieved for 10 μm particles, as well as fluid parcels of the original stream when collecting different cross-sectional fractions of the flow. Segments of the flow that were collected in different outlets and analysed off-chip are indicated. (d) Stream splitting. (e) Microfluidic mixing (Pe~4 × 104,Re=20). All the flows ina–eoperate atRe=20, Scale bars, 50 μm. Figure 5: Applications of fluid flow programming. ( a ) Extraction of particles from a fluid stream. While the fluid moves away from the channel centre due to inertial effects, particles are maintained at the channel centerline due to inertial focusing. ( b ) Separation of particles by size using a similar geometry (10 μm particles remain focused while 1 μm particles follow fluid streams). ( c ) Moving fluid streams and solution exchange around particles. High extraction yield (>95%) with high purity (>90%) is achieved for 10 μm particles, as well as fluid parcels of the original stream when collecting different cross-sectional fractions of the flow. Segments of the flow that were collected in different outlets and analysed off-chip are indicated. ( d ) Stream splitting. ( e ) Microfluidic mixing ( Pe ~4 × 10 4 , Re =20). All the flows in a – e operate at Re =20, Scale bars, 50 μm. Full size image The ability to engineer fluid flows in channels—particularly controlling cross-sectional shape and rotating and moving fluid streams—introduces a fundamental new capability potentially useful in a variety of other applications. Controlling the cross-sectional shape of a monomer stream enables manufacture of new classes of polymerized fibres with engineered interactions (for example, interlocking or self-assembling fibre materials) [8] , [24] , [25] , [26] , [27] , [28] . By combining this cross-sectional shape control of a polymer pre-cursor stream with optical patterning transverse to the flow direction [6] , [7] fabrication of an infinite set of truly three-dimensional particle shapes would be possible. Additionally, engineering a variety of cross-sectional lens shapes with a fluid of separate index of refraction [29] can be of use for opto-fluidic control and sensing [30] . Rotating or moving fluid streams to be analysed away from walls to regions of uniform downstream velocity at the channel centre can minimize Taylor dispersion [9] , bring fluid into a small focal spot for optical interrogation [31] , [32] or reduce fouling and adhesion to channel surfaces. Conversely, bringing fluid to narrow slow moving regions near channel walls can enhance surface reactions (for example, immunoassays [33] ), or aid in affinity capture of cells [34] or molecules. Additionally, utilizing this platform to deterministically guide liquid in microchannels can enhance heat transfer, especially in electronic cooling, by maximizing the efficiency of coolant usage near hot spots and enabling the usage of larger channels with lower pressure drops and power consumption in these systems [35] , [36] , [37] . We anticipate these future applications will be enabled as the complexity of available functions increases or the inverse problem to produce a desired sculpted flow shape is solved computationally, aided by the limited set of transformations which do not require full fluid dynamic simulations for each tested sequence. A growth in flow shape complexity and control with time could be expected, as for computational programming, because no expert knowledge of hardware is needed and operations are abstracted and assembled in an easily communicated form. Microfabrication Microfluidic devices were fabricated using polydimethylsiloxane (PDMS) replica moudling processes [38] . Briefly, standard lithographic techniques were used to produce a mold from a silicon master spin-coated with SU-8 photoresist (MicroChem Corp.). PDMS chips were produced from this mold using Sylgard 184 Elastomer Kit (Dow Corning Corporation). Inlet and outlet holes were punched through PDMS using a pin vise (Technical Innovations, Inc.). PDMS and glass were activated by air plasma (Plasma Cleaner, Harrick Plasma) and bonded together to enclose the channels. In order to see the PDMS walls of the channel ( Fig. 1b ) Rhodamine B red dye, which permeates PDMS, was infused into the channel and washed before the experiments. Dye and bead suspensions To help visualization, the fluid stream was mixed with fluorescein isothiocyanate dextran 500 kDa (4 μM in deionized water) or with blue food dye. Fluorescent monodisperse particles (1 μm and 10 μm, 1.05 g ml −1 ) were purchased from Duke Scientific. Particles were mixed in deionized water. Fluid streams and particle suspensions were pumped into the devices through PEEK tubing (Upchurch Scientific Product No. 1569) using a syringe pump (Harvard Apparatus PHD 2000). Imaging Confocal imaging was performed at the California NanoSystems Institute using a Leica inverted SP1 confocal microscope. Confocal images are the average of 8 y-z scans. Fluorescent images were recorded using a Photometrics CoolSNAP HQ2 CCD (charge-coupled device) camera mounted on a Nikon Eclipse Ti microscope. Images were captured with Nikon NIS-Elements AR 3.0 software. For high-precision observations and measurements, high-speed images were also recorded using a Phantom v7.3 high-speed camera (Vision Research Inc.) and Phantom Camera Control software. Numerical simulations for phase diagram The numerical simulations were performed using an in-house, parallel framework based on stabilized finite element methods. The phase diagram was built by performing more than 2,200 of these numerical simulations with different configurations. This was automated using a novel fault tolerant strategy that deployed the finite element framework across high performance computing clusters (NSF XSEDE: Ranger system and Iowa State: Cystorm system). Lateral velocity field arrow plot creation The arrow plots presented in the manuscript show the net rotational flow that is occurring near a pillar, which means that it is extracted by the comparison of the lateral position of fluid parcels between the inlet and outlet. Each arrow indicates the net lateral velocity at that position in the channel cross-section. ‘Net lateral velocity’ is defined for each fluid parcel as the average lateral velocity of the fluid parcel as it travels downstream, from the inlet to the outlet. It is numerically calculated by dividing the total lateral displacement of a fluid parcel (that has travelled from inlet to the outlet) by the total time taken for this motion to occur. Definition of σ In order to quantitatively compare the amount of lateral fluid motion for different flow and geometric conditions we define a normalized value, σ . It is defined as the mean of the net lateral velocities (described above) at z =0 (middle-height of the channel), normalized by the average downstream velocity of the main flow, in other words. This is essentially a measure of the distance fluid has moved laterally (on average and at the channel mid-plane) per unit of length it travels downstream. How to cite this article: Amini, H. et al. Engineering fluid flow using sequenced microstructures. Nat. Commun. 4:1826 doi: 10.1038/ncomms2841 (2013).